Quantum state majorization at the output of bosonic Gaussian channels Quantum communication theory explores the implications of quantum mechanics to the tasks of information transmission. Many physical channels can be formally described as quantum Gaussian operations acting on bosonic quantum states. Depending on the input state and on the quality of the channel, the output suffers certain amount of noise. For a long time it has been conjectured, but never proved, that output states of Gaussian channels corresponding to coherent input signals are the less noisy ones (in the sense of a majorization criterion). Here we prove this conjecture. Specifically we show that every output state of a phase-insensitive Gaussian channel is majorized by the output state corresponding to a coherent input. The proof is based on the optimality of coherent states for the minimization of strictly concave output functionals. Moreover we show that coherent states are the unique optimizers. Design and analysis of the optimal protocols for processing, storing and transmitting information is the subject of the fundamental research field of information theory pioneered in the last century by C. E. Shannon [1] . In reality, information needs to be recorded necessarily onto a physical medium and transmitted via a physical channel. Therefore, in addition to information theory, communication protocols should obey the laws of physics. The progress in microminiaturization of data-processing systems leads to use of information carriers that cannot be described by a classical theory and behave according to quantum mechanics (for example, photons, electrons, atoms, etc.). The task of quantum information and communication theory is to study the laws of information transmission and processing in quantum mechanical systems [2] , [3] , [4] , [5] . A large part of quantum communication theory is devoted to the transmission of electromagnetic radiation via bosonic Gaussian channels [4] , [6] , [7] , [8] . The latter are formally defined as completely positive and trace preserving operations mapping Gaussian input states into Gaussian output states. The most relevant channels are also invariant under phase space rotations and are called phase-insensitive. For example, the transmission of optical quantum states through realistic physical devices [3] (like for example, optical fibres, free space communication lines, dielectric media, etc.) can be described by phase-insensitive Gaussian channels. In the spirit of classical communication theory [1] , one may ask what is the minimum amount of ‘disorder’ achievable at the output of a Gaussian channel. For quantum systems there are two main figures of merit which can be used to quantify the idea of disorder [9] , [10] , [11] , [12] : the von Neumann entropy and the concept of majorization. The entropy of a state ρ is defined as S ( ρ )=−Tr[ ρ log( ρ )] and one can say that a state ρ 1 is more disordered than ρ 2 if S ( ρ 1 )> S ( ρ 2 ). A different (and stronger) way of saying that ρ 1 is more disordered than ρ 2 is given by the following equation: where the vectors and consist of the eigenvalues of the respective states arranged in decreasing order. If the condition (1) is satisfied then one says that ρ 2 majorizes ρ 1 and this is usually indicated by the expression ρ 2 ρ 1 . The previous definition has a very intuitive operational interpretation since it can be shown that ρ 2 ρ 1 if and only if ρ 1 can be obtained from ρ 2 by a proper convex combination of unitary operations [9] , [10] , [11] , [12] . These considerations extend also to the infinite-dimensional case [13] relevant for the quantum description of electromagnetic modes. According to the previous ideas of disorder, for a phase-insensitive bosonic Gaussian channel it was conjectured [14] that: (1) the minimum-output entropy is achieved by coherent input states, (2) the output states resulting from coherent input states majorize all other output states. A graphical representation of the last property is given in Fig. 1 . Both conjectures have broad implications in many research areas like classical and quantum optics, telecommunication engineering, mathematical and statistical physics, and for this reason they attracted the attention of many scientists. In particular, the validity of conjecture (1) and (2) has a number of important corollaries and relations ranging from entanglement theory [15] , [16] , [17] , [18] , channel capacities [6] , [14] , [18] , [19] , [20] , [21] , [22] , entropic inequalities [19] , [20] , [23] , [24] to quantum discord [25] , [26] . 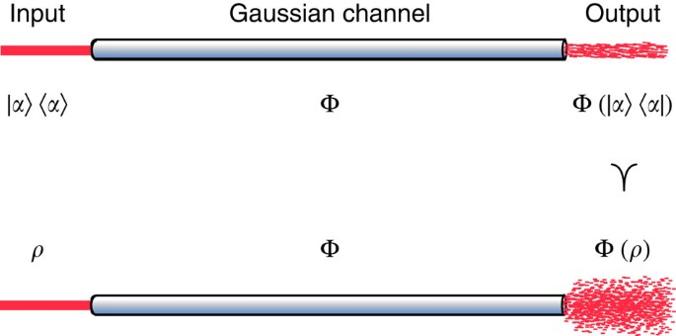Figure 1: Graphical representation of the majorization conjecture (2). A coherent state |α› ‹α| and an arbitrary stateρare both transmitted through the same phase-insensitive Gaussian channel Φ. The respective output states always satisfy the majorization relation Φ(|α› ‹α|)Φ(ρ). This means that coherent input states produce less ‘noise’ at the output of the communication channel. Figure 1: Graphical representation of the majorization conjecture (2). A coherent state | α › ‹ α | and an arbitrary state ρ are both transmitted through the same phase-insensitive Gaussian channel Φ. The respective output states always satisfy the majorization relation Φ(| α › ‹ α |) Φ( ρ ). This means that coherent input states produce less ‘noise’ at the output of the communication channel. Full size image In the last decade, many analytical and numerical evidences supporting both conjectures were presented [14] , [19] , [20] , [21] , [22] , [23] , [24] , [27] , [28] , [29] , [30] , [31] but a general proof was missing. Only very recently the first one was finally proved [18] , [32] under the assumption of a finite mean energy. In this work we prove the second conjecture (2) and highlight some of its implications. Moreover it is easy to show that ρ 2 ρ 1 implies S ( ρ 1 )≥ S ( ρ 2 ), therefore the statement (2) is stronger than the conjecture (1) and the result presented in this work can also be seen as a proof of the minimum-output entropy conjecture, without any energy constraint. Thus both gaps in the theory are now definitely closed. Gaussian channels Every quantum channel [4] , [33] can be described as a global unitary operation applied to the tensor product of the state of the system ρ S and the state of an appropriate environment ρ E : Single-mode phase-insensitive channels [21] can be classified in three main classes , n and . Physically, represents a thermal channel, which can be realized by a beamsplitter of transmissivity, η , mixing the input signal with a thermal state, ρ E , with mean photon number, N : where a and a E are the annihilation operators of the system and of the environment, respectively. Then, n is the classical additive noise channel where the input state is displaced according to a random Gaussian distribution of variance n and, finally, is the quantum amplifier where the state of the environment is in a thermal state ρ E : More precisely, these channels can be defined according to their action on the quantum characteristic function in the following way [8] : Any of the previous phase-insensitive channels, which we denote by the symbol Φ, can always be decomposed [22] , [32] into a pure-loss channel followed by a quantum-limited amplifier: for appropriate values of κ and η . In what follows we will make use of this decomposition and for simplicity we introduce the symbols k and η for indicating the respective quantum-limited channels with N =0. Complementary channels One can associate to every channel (2) the respective complementary channel defined as and physically representing the flow of information from the input state to the environment [4] , [8] . An important property of complementary channels is that, whenever the system and the environment are in a pure state, the nonzero spectra of the output states Φ(| ψ S › ‹ ψ S |) and are equal. This is a simple consequence of the Schmidt decomposition of the global pure state (for an explicit proof see ref. 33 ). In what follows the complementary channel of the quantum-limited amplifier will play an important role. In this case ρ E is the vacuum and U is the two-mode squeezing operation [8] acting in the Heisenberg picture according to equation (4) and From equation (4), tracing out the environment, one obtains k defined in equation (7) with N =0. From equation (10) instead, tracing out the system, we get the complementary channel acting on the characteristic function as Importantly, the complementary channel does not have the same structure as the amplifier given in equation (7), since the complex variable μ appears conjugated in the RHS of equation (11). In quantum optics this effect is known as phase conjugation or time reversal and corresponds to the positive (but not completely positive) map which at the level of density operators behaves as transposition T ( ρ )= ρ T in the Fock basis and therefore it preserves the eigenvalues. This means that each time we are interested in spectral properties of the output state (as in the proof of Lemma 1), we can neglect the effect of the phase conjugation operator T . Minimization of strictly concave functionals Before giving the proof of the majorization conjecture we consider an important minimization problem. Let F : → be a unitary invariant and strictly concave functional acting on the infinite-dimensional Hilbert space of density matrices of a single bosonic mode. We assume that F can take values in [0, +∞], having in mind applications to the von Neumann entropy. Unitary invariance means that F ( UρU † )= F ( ρ ) for every unitary matrix U , while strict concavity means that and the equality is obtained only for ρ 1 = ρ 2 . The problem that we want to address is the minimization of such functionals at the output of a phase-insensitive channel, where the optimization is performed over all possible input states: An important case is when the functional is replaced by the von Neumann entropy F ( ρ )= S ( ρ )=−Tr[ ρ log( ρ )], and the minimization problem reduces to the minimum-output entropy conjecture (1) [14] , [30] . We recall that this conjecture claims that the minimum is achieved by input coherent states of the form and was recently proved [32] . With the next lemma, we are going to show that this extremal property of coherent states is more general and can be applied to every functional of the kind that we have previously introduced. Lemma 1 : Let Φ be a phase-insensitive bosonic channel. Then, for every non-negative unitary invariant and strictly concave functional, F, and for every quantum state, ρ , we have where | α › is any coherent state. Moreover the equality is achieved only if ρ is a coherent state. Proof : for a pure-loss channel , the proof is simple. Indeed coherent states are mapped to pure coherent states under the action of . Since F is concave and unitary invariant, when applied to pure states it necessarily achieves its minimum. So, in this case, inequality (16) is satisfied (the uniqueness property of coherent states is considered in the last part of this proof and is a consequence of Lemma 2 of the Methods section). For a general phase-insensitive channel Φ we can use the decomposition of equation (8). A direct consequence of this decomposition is that we just need to prove the lemma for the minimal-noise amplification channel Φ= κ since coherent states remain coherent after a beam splitter. Let be the conjugate channel of κ . Again, can be itself decomposed according to the structure of equation (8). Indeed, from a direct application of equations (7, 11, 12) one can verify that where T is the phase conjugation operator and η =1−1/ κ . Let be the set of all pure input states minimizing the functional F at the output of the channel κ . We need to show that coincides the set of coherent states. Let us take an optimal state | ψ › ε . From the property of complementary channels and of the phase conjugation operator mentioned before we have that, κ (| ψ › ‹| ψ |), and have the same spectrum. Since F is unitary invariant, it necessarily depends only on the eigenvalues and we have . Therefore, where {| ψ j › } is the ensemble of states obtained after the beam splitter: From the concavity of F we have By hypothesis | ψ › ε and so F [ κ ( ψ › ‹ ψ |)]≤ F [ κ ( ψ j › ‹ ψ j |)] for each j . This can be true only if the inequality (19) is saturated and, from the hypothesis of strict concavity, we get From the definition of the quantum amplifier given in equation (7), it is evident that equal output states are possible only for equal input states: | ψ j › =| ψ ′› for every j . As a consequence equation (18), reduces to But now comes into play an important property of the beamsplitter which is known from the field of quantum optics [34] , [35] , [36] , namely that only coherent states remain pure under the action of a beamsplitter (Lemma 2 in the Methods section). Therefore, since equation (21) is valid for every choice of | ψ › ε , then necessarily contains only coherent states. Moreover, for every Gaussian channel a displacement of the input state corresponds to a (possibly different) displacement of the output state [7] , [8] , which obviously does not change the entropy. Since coherent states are equivalent up to displacement operations it means that coincides with the whole set of coherent states. Majorization at the output of the channel We can finally state our main result which proves the validity of the majorization conjecture (2). A graphical representation of this property is given in Fig. 1 . Proposition 1 : Let Φ be a phase-insensitive bosonic channel. Then, for every input state ρ , where | α › is any coherent state. Proof : Let be the class of real non-negative strictly concave functions f defined on the segment [0, 1]. Consider the following functional where f ε . Then F is well-defined with values in [0, +∞], since all the terms in the series are non-negative. Moreover, it is unitary invariant and it can be shown that the strict concavity of f as a function of real numbers implies the strict concavity of F with respect to quantum states [12] . Therefore the previous lemma can be applied and we get, for every state ρ and every strictly concave function f , A well-known theorem [9] , [10] , [11] in the finite dimensional case states that ρ 2 ρ 1 if and only if for every concave function f . Moreover, a similar result is valid also for strictly concave functions f ε and in infinite dimensions (see Lemma 3 in the Methods section). This concludes the proof. As a final remark, as the von Neumann entropy is a strictly concave functional [11] , we get an alternative proof (with respect to the one given in ref. 32 ) of the minimal-output entropy conjecture. By applying Lemma 1 with the choice F ( ρ )=−Tr[ ρ log( ρ )], we get a slightly stronger version of the conjecture (1): the minimum output entropy of a phase-insensitive channel is achieved only by coherent input states. Notice that, differently from the proof presented in ref. 32 , this result does not require the assumption that the mean energy of the input should be finite and proves also that coherent states are the unique optimizers. Moreover, choosing f ( x )= x − x p , p >1, leads to the proof of the similar statement for the minimal-output Renyi entropies of all orders p >1. The main result of this paper is that every output state of a phase-insensitive bosonic Gaussian channel is majorized by the output associated to a coherent input state (proof of the majorization conjecture). We also prove that coherent input states are the unique minimizers of arbitrary non-negative strictly concave output functionals and, in particular, of the von Neumann entropy (minimum-output entropy conjecture). As compared with the proof of the minimal output entropy conjecture given in ref. 32 , our result does not require the finiteness of the mean energy and proves the uniqueness of coherent states. Our work, while closing two longstanding open problems in quantum communication theory, has a large variety of implications and consequences. For example, by using Lemma 1 and Proposition 1 one can: compute the entanglement of formation of non-symmetric Gaussian states (see the last section of ref. 18 ), evaluate the classical capacity of Gaussian channels [18] and compute the exact quantum discord [25] for a large class of channels [26] . Moreover, from Proposition 1, we conclude that coherent input states minimize every Schur-concave output function like Renyi entropies of arbitrary order [19] , [20] , [23] , [24] . Finally, it is a simple implication that the pure entangled state |Ψ out › obtained from a unitary dilation of a phase-insensitive Gaussian channel is more entangled than the output state |Ψ out › ′ obtained with a coherent input. What is more, from the well-known relationship between entanglement and majorization [9] , we also know that |Ψ out › ′ can be obtained from |Ψ out › with local operations and classical communication. The previous facts are just some important examples while a detailed analysis of all the possible implications will be the subject of future works. Some useful facts To make our analysis self-contained, in this section we present two properties (Lemma 1 and Lemma 2), which are used in the proof of the majorization conjecture. Lemma 2 : Coherent states are the only input pure states which produce a pure output for a beamsplitter. This property is more or less implicit in several quantum optics papers [34] , [35] , [36] . Here we present a complete proof, following an argument similar to one used in ref. 34 , but using the formalism of quantum characteristic functions. Proof : Let be the beamsplitter of transmissivity η , 0< η <1, and Then the complementary channel, which is the beamsplitter of transmissivity 1− η satisfies a similar relation as the outputs of complementary channels have identical nonzero spectra. Therefore we have where U is the unitary implementing the minimal dilation of η . The corresponding canonical transformation of the annihilation operators a , a E for the system and the environment is and the environment mode a E , a E † is in the vacuum state. In phase space, this produces a symplectic transformation in the variables of the characteristic functions: By letting z E =0 and z =0, respectively, we obtain Thus, after the change of variables , and denoting , we get The function ω ( z ), as well as the characteristic function χ ( z ), is continuous and satisfies . The only solution of equation (33) satisfying these conditions is the exponential function for some complex α . Thus we obtain which is the characteristic function of a coherent state | α › . Lemma 3 : Given two (finite or infinite dimensional) vectors λ and λ ′ whose elements are non-negative and normalized , the following two relations are equivalent: for every function f ε , where is the class of real non-negative strictly concave functions defined on the segment [0, 1]. Proof : It is well-known in finite-dimensional majorization theory [9] , [10] , [11] , [12] that if λ ′ λ then inequality (36) is satisfied for every concave function and so, in particular, for strictly concave functions. From the infinite dimensional generalization of the Horn–Schur theorem [13] one can extend this result to all functions f ε , using the fact that the two series appearing in inequality (36) converge unconditionally to a value in [0, +∞]. To prove the converse implication suppose that the majorization relation (35) is not valid, then we construct an f ε which violates the condition (36). As shown in ref. 11 , a simple concave (but nonstrictly concave) function can be found in a constructive way by using the following ansatz: If λ′ λ then there exists a smallest integer n for which . It is easy to show [11] that, by choosing , the function f 0 violates the condition (36), that is, there is a positive and finite δ such that However, this does not conclude our proof because f 0 is not strictly concave. For this reason we take a slightly different function which is strictly concave for every ∈ >0 and belongs to the class . Now, for an arbitrary vector λ , by using the positivity and the normalization of the elements { λ i } we get the following convergence: From the last continuity relation together with equation (38) we get: The last term can be made positive by choosing ∈ < δ . Summarizing, we have shown that whenever the majorization relation (35) is not satisfied, there exists a small but finite ∈ such that f ∈ violates the inequality (36). Therefore the two conditions equation (35) and equation (36) are equivalent. How to cite this article: Mari, A. et al. Quantum state majorization at the output of bosonic Gaussian channels. Nat. Commun. 5:3826 doi: 10.1038/ncomms4826 (2014).